Humangephyrinis encompassed within giant functional noncoding yin–yang sequences Gephyrin is a highly conserved gene that is vital for the organization of proteins at inhibitory receptors, molybdenum cofactor biosynthesis and other diverse functions. Its specific function is intricately regulated and its aberrant activities have been observed for a number of human diseases. Here we report a remarkable yin–yang haplotype pattern encompassing gephyrin . Yin–yang haplotypes arise when a stretch of DNA evolves to present two disparate forms that bear differing states for nucleotide variations along their lengths. The gephyrin yin–yang pair consists of 284 divergent nucleotide states and both variants vary drastically from their mutual ancestral haplotype, suggesting rapid evolution. Several independent lines of evidence indicate strong positive selection on the region and suggest these high-frequency haplotypes represent two distinct functional mechanisms. This discovery holds potential to deepen our understanding of variable human-specific regulation of gephyrin while providing clues for rapid evolutionary events and allelic migrations buried within human history. Gephyrin is a 93-kDa multi-functional protein that was named after the Greek word for ‘bridge’ due to its role in linking neurotransmitter receptors to the microtubule cytoskeleton. It binds polymerized tubulin with high affinity, probably due to a motif with high sequence similarities to the binding domains of MAP2 and Tau [1] , [2] . This protein dynamically provides a scaffold for clustering of proteins for both glycine and GABA-A receptors in inhibitory synapses, plays a crucial role in synapse formation and plasticity, and is believed to hold a central role in maintaining homeostatic excitation–inhibition balance [3] . Gephyrin has remarkably diverse functions. It associates with translation initiation machinery and has been implicated in the regulation of synaptic protein synthesis [4] . It also interacts with mammalian target of rapamycin (mTOR), a key protein for nutrient-sensitive cell cycle regulation, and has been shown to be required for downstream mTOR signalling [5] . Interestingly, gephyrin clustering at GABAergic synapses is increased by brain-derived neurotrophic factor-mediated mTOR activation and decreased by glycogen synthase kinase 3β phosphorylation [6] . Gephyrin is also indispensable for molybdenum cofactor (MoCo) biosynthesis, as it is necessary for the insertion of molybdenum during this essential process [3] . MoCo deficiency leads to severe neurological damage and early childhood death. The fusion of an ancient function (MoCo biosynthesis) with an evolutionarily young function (neuroreceptor clustering) is believed to have an impact on catalytic efficacy of MoCo synthesis by improving product–substrate channelling [7] . Finally, gephyrin was recently observed to localize within a ~600-kDa cytoplasmic complex of unknown composition in non-neuronal cells, and it has been speculated that this complex might be involved in nutrient sensing, glucose metabolism or ageing, perhaps due to gephyrin’s interactions with mTOR [8] . Gephyrin ’s protein-coding regions are identical to the chimpanzee orthologue and are highly conserved across species. In contrast, regulation of this gene is highly variable. Gephyrin produces complex alternative splicing isoforms, which are crucial for its diverse functions, and at least 8 of the 29 exons of this mosaic gene are subject to alternative splicing in species-, tissue-, cell- and/or environmentally specific manners [1] , [9] , [10] , [11] , [12] , [13] . It is believed that the gephyrin scaffold in inhibitory synapses is a hexagonal lattice with twofold and threefold symmetry, and some alternative splicing isoforms disrupt this structure [14] . These alternate forms may provide a mechanism for plasticity and the dynamics of receptor anchoring by acting as dominant-negative variants, which bind and remove receptors from synapses [14] . In concordance, MoCo biosynthesis activity is also isoform dependent, with various cassette insertions or deletions inactivating this synthesis [15] . For these reasons, unravelling the regulatory mechanisms is essential for elucidating and understanding gephyrin’s dynamic and diverse activities and functions. Markers within introns and in close genomic proximity are prominent candidates for regulatory elements and the region encompassing gephyrin has been noted previously by two different groups. A 2.1-Mb region of homozygosity (ROH) in this location was discovered in 2010 (ref. 16 ). ROHs are correlated with linkage disequilibrium (LD) and have been observed to sometimes bear markedly disparate haplotypes [17] . In their 2010 paper, Curtis and Vine [16] determined 20 genomic regions that had the largest number of subjects showing an ROH and studied the haplotypes of the 9 single-nucleotide polymorphisms (SNPs) at the centre of each of these regions, observing that the haplotypes showed significant excess disparity, that is, a tendency for pairs to simultaneously differ at multiple SNPs. The term yin–yang haplotypes was coined to capture the polarity of such structures when a 24-SNP pattern for which two haplotypes with differing states at each site and a combined frequency of 0.50 was discovered by Zhang et al . [18] Curtis and Vine [16] noted that the ten most common haplotypes for the nine SNPs in the gephyrin region had a combined frequency of 0.67, indicating surprisingly little diversity of haplotypes. Interestingly, eight of these ten haplotypes yielded four pairs of yin–yang haplotypes, each of which bore different allelic states at all nine SNPs, indicating the haplotypes which did occur were remarkably different from each other. In a 2012 study unrelated to yin–yang haplotypes, this region was identified by Park [19] in a genome-wide scan of LD. This study identified an exceptionally strong LD block and discussed ‘extraordinary’ frequency spectra for all HapMap [20] populations in a 1-Mb region centred on intron 2 of gephyrin . Park concluded that the phenomenon could be due to a selective sweep and reviewed a number of selective pressure analyses, noting that this region had been included in Supplementary Materials by two of these studies [21] , [22] and completely overlooked by the others. Park [19] noted the uniqueness of this region, but the underlying yin–yang pattern went undetected. In an exploration of genome-wide population data, we apply a recently developed method named BlocBuster [23] to SNP data for individuals in HapMap [20] populations and discover a high-frequency 284-SNP yin–yang haplotype pair embedded in noncoding regions within and surrounding gephyrin . Both haplotypes vary drastically from their mutual ancestral haplotype, yet they are highly conserved across global human populations, specifying two radically distinct evolutionary paths within a single genomic region. Furthermore, we report several independent lines of evidence indicating the identified yin and yang haplotypes are under selective pressure, thereby suggesting two distinct and functionally significant mechanisms underlie these regions. Gephyrin is encompassed within a yin–yang haplotype pair We applied our BlocBuster method [23] (see Methods) to SNP data for unrelated individuals in four HapMap populations [20] : Northern and western European ancestry (CEU), Han Chinese in Beijing, China (CHB), Japanese in Tokyo (JPT) and Yoruba in Ibadan, Nigeria (YRI). BlocBuster constructs networks that reveal haploid groups of SNP alleles that are inter-correlated, referred to as blocs . The results were highly consistent across all of the autosomal chromosomes, except chromosome 14, which had unusual network characteristics ( Supplementary Note 1 ). We then applied BlocBuster to HapMap data for four different populations: Gujarati Indians living in Houston, USA (GIH), Luhya in Webuye, Kenya (LWK), Maasai in Kinyawa, Kenya (MKK) and Toscani in Italia (TSI) [20] , and again chromosome 14 was an outlier. A closer examination revealed the source of the anomalies—73% of all of the edges in the first network were concentrated into a single bloc with 255 SNP alleles and 74% of the edges in the second network were concentrated into 2 blocs with 264 and 257 SNP alleles, respectively. The two blocs in the second network share 241 SNPs in common, with opposite alleles appearing in each bloc. Furthermore, these SNPs span the same genomic region as the bloc in the first network. Overall, the three blocs found by the two analyses capture a single yin–yang haplotype pair. The three blocs possess 226 SNPs in common and span across 284 unique SNPs overall ( Supplementary Data Set 1 ). We define this yin–yang pair using these 284 highly correlated SNPs. (See Supplementary Note 1 and Supplementary Fig. 1 for description of an additional bloc corresponding to the yang haplotype for the first analysis.) This yin–yang pair is located on 14q23.3, encompassing gephyrin ( GPHN ) and extending beyond by ~300 kb upstream and downstream of gephyrin ( Fig. 1 ). Interestingly, all of the divergent markers appear within introns, long noncoding RNA, or intergenic regions. As illustrated by the colour-coded bar above the first two columns of matrices in Fig. 1 , few SNPs are downstream from gephyrin (2.%, 3.4% and 5.1% for the 255-, 264- and 257-SNP blocs, respectively) and none lie within MPP5 . About one-fifth of the SNPs lie upstream from gephyrin (19.2%, 18.6% and 20.6%) and all three blocs include the same eight SNPs within the long noncoding RNA, LINC00238 . Most of the SNPs lie within noncoding regions of gephyrin (78.0%, 78.0% and 74.3%). 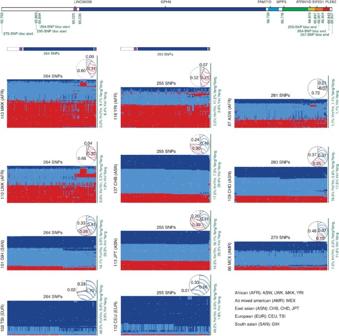Figure 1: Yin–yang haplotypes. (Best viewed in colour, high-resolution image available online asSupplementary Fig. 3). Upper panel: yin–yang region with colour-coded genes and positions in kb. Lower panel: genotypes for the yin–yang haplotypes. The first column of matrices represents the ‘yin’ bloc identified in the analysis of the GIH, LWK, MKK and TSI populations. The middle column represents the ‘yin’ bloc from the CEU, CHB, JPT and YRI analysis. The last column represents the available yin–yang SNPs for each of the three additional HapMap populations: ASW, CHD and Mexican ancestry in Los Angeles, California. For each matrix, each column represents an SNP and each row represents an individual (rows are rearranged to place similar individuals near each other). Colour-coded bars at the top of the first two columns indicate SNP positions by matching the gene colour from the top panel. Dark blue indicates homozygote for SNP allele in the bloc, red for homozygote for alternate allele, light blue for heterozygote and white for missing data. A solid dark blue horizontal line represents an individual that possesses two yin haplotypes and a solid red line represents a yang homozygote. Percentages of individuals that are homozygotes or heterozygotes for the yin and yang haplotypes are shown on the right side of each matrix. Yin (blue) and yang (red) haplotype frequencies are shown in pie chart above each matrix, with white indicating the percentage of haplotypes that are not 100% yin nor 100% yang. Figure 1: Yin–yang haplotypes. (Best viewed in colour, high-resolution image available online as Supplementary Fig. 3 ). Upper panel: yin–yang region with colour-coded genes and positions in kb. Lower panel: genotypes for the yin–yang haplotypes. The first column of matrices represents the ‘yin’ bloc identified in the analysis of the GIH, LWK, MKK and TSI populations. The middle column represents the ‘yin’ bloc from the CEU, CHB, JPT and YRI analysis. The last column represents the available yin–yang SNPs for each of the three additional HapMap populations: ASW, CHD and Mexican ancestry in Los Angeles, California. For each matrix, each column represents an SNP and each row represents an individual (rows are rearranged to place similar individuals near each other). Colour-coded bars at the top of the first two columns indicate SNP positions by matching the gene colour from the top panel. Dark blue indicates homozygote for SNP allele in the bloc, red for homozygote for alternate allele, light blue for heterozygote and white for missing data. A solid dark blue horizontal line represents an individual that possesses two yin haplotypes and a solid red line represents a yang homozygote. Percentages of individuals that are homozygotes or heterozygotes for the yin and yang haplotypes are shown on the right side of each matrix. Yin (blue) and yang (red) haplotype frequencies are shown in pie chart above each matrix, with white indicating the percentage of haplotypes that are not 100% yin nor 100% yang. Full size image Owing to the high proportion of heterozygotes within the Asian populations, we further interrogated these results using computationally phased haplotypes for the CHB and JPT populations provided by the HapMap Consortium. There are few yin–yang SNPs downstream from gephyrin and they are sparser and more variable than the other SNPs; hence, we omitted them from this analysis (see Methods). The available phased haplotypes did not include all of the yin–yang SNPs, and after removing SNPs with >5% missing data there remained 236 SNPs in phased haplotypes for 170 CHB+JPT individuals, for a total of 340 phased chromosomes. 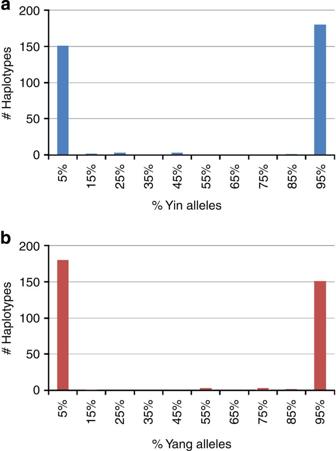Figure 2: Haplotype compositions. The numbers of CHB and JPT phased chromosomes possessing various percentages of (a) yin and (b) yang SNP alleles are shown. As these are biallelic SNPs, the plots are mirror images (for example, the haplotypes representing the 0%–10% range inaare the same haplotypes representing the 90%–100% range inb). Only 9 of the 340 phased chromosomes lie in the 10%–90% range for yin or yang alleles. Figure 2 shows the percentages of yin and yang SNP alleles found on each of the 340 phased chromosomes. These plots illustrate the prominence of the two divergent haplotypes and rarity of intermediate haplotypes. Figure 2: Haplotype compositions. The numbers of CHB and JPT phased chromosomes possessing various percentages of ( a ) yin and ( b ) yang SNP alleles are shown. As these are biallelic SNPs, the plots are mirror images (for example, the haplotypes representing the 0%–10% range in a are the same haplotypes representing the 90%–100% range in b ). Only 9 of the 340 phased chromosomes lie in the 10%–90% range for yin or yang alleles. Full size image Interleaving SNPs lying between the yin–yang SNPs generally have low minor allele frequencies, as shown in Fig. 3 and Supplementary Figs 4–11 . A close examination of the interleaving SNPs for the Asian populations indicate that a handful of individuals tend to possess most of the minor alleles (appearing in the high-resolution images as horizontal dotted lines across the yin–yang region of the matrix). Note that these individuals are not correlated with yin or yang haplotype status and consequently the variants are not likely to be hitchhiking with the yin or yang haplotypes. 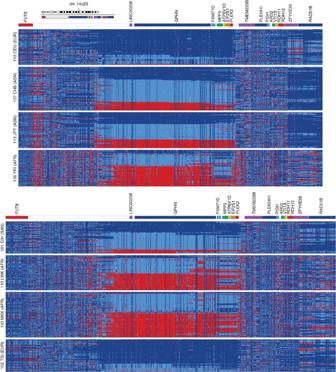Figure 3: All SNPs within and surrounding the yin–yang region. The available HapMap SNPs within the yin–yang region (355 for the first four populations and 436 for the second four populations) are shown, along with 300 SNPs upstream and 300 downstream. (Best viewed in colour; seeFig. 1caption for details.) Homozygotes in the minor allele for the CEU or TSI populations are coloured red, heterozygotes are light blue, homozygotes in the alternate allele are dark blue and missing data are white. SNPs with low minor allele frequencies (MAF) appear as vertical columns that are predominantly either dark blue or red. Colour bars above each group indicate the distributions of the SNPs across genomic regions. High-resolution images are available online asSupplementary Figs 4–11. Figure 3: All SNPs within and surrounding the yin–yang region. The available HapMap SNPs within the yin–yang region (355 for the first four populations and 436 for the second four populations) are shown, along with 300 SNPs upstream and 300 downstream. (Best viewed in colour; see Fig. 1 caption for details.) Homozygotes in the minor allele for the CEU or TSI populations are coloured red, heterozygotes are light blue, homozygotes in the alternate allele are dark blue and missing data are white. SNPs with low minor allele frequencies (MAF) appear as vertical columns that are predominantly either dark blue or red. Colour bars above each group indicate the distributions of the SNPs across genomic regions. High-resolution images are available online as Supplementary Figs 4–11 . Full size image These results indicate exceptionally high linkage among the 284 SNPs spanning more than 1 Mb and primarily located within noncoding regions of gephyrin and immediately upstream. Notably, two distinct haplotypes with differing states at all of the SNPs are unusually common and appear across global populations. Conservation of yin–yang haplotypes within Homo populations As shown in Fig. 1 , the yin and yang haplotypes are prominent for all 11 HapMap populations, with combined frequencies ranging from 0.28 to 0.80. The pie charts in Fig. 1 indicate the frequencies of the yin and yang haplotypes, and the white regions represent the portion of partial haplotypes with one or more alleles that do not conform to an entire yin or yang pattern. The percentages of homozygotes and heterozygotes are listed on the right of each matrix. The two European-ancestry populations, CEU and TSI, have large percentages of yin homozygotes. Three African populations, LWK, MKK and YRI, have high frequencies of the yang haplotypes and possess a recombination block near the end of the haplotypes, while individuals with African ancestry in Southwest USA (ASW) have a yang frequency of 0.07 and a shorter recombination block. The East and South Asian populations (CHB, Chinese in Metropolitan Denver, Colorado, USA (CHD), GIH and JPT) exhibit the strongest mix of yin and yang haplotypes. Every one of these four populations exhibit frequencies of at least 0.25 for each of the yin and yang haplotypes, and the combined frequencies for the CHB and JPT populations reach 0.76 and 0.80, respectively. The CHD are similar to the CHB, although there is some recombination near the start of the haplotypes for the CHD. The GIH, with ancestry from the Indian subcontinent, possess frequencies that are similar to the East Asian populations, albeit with decreased yang homozygotes and increased haplotype diversity. The 1000 Genomes Project [24] includes genotype data for 2,504 individuals from 26 global populations, representing each major human ancestry. Although imputed data are included in these files, we built a BlocBuster network to test the robustness of the results found for the HapMap data, as described in Supplementary Note 2 . The yin and yang haplotypes are pronounced for these individuals ( Supplementary Fig. 2 ), thereby supporting the HapMap results. Ancestral alleles for the 284 yin–yang SNPs were determined by comparing human and chimpanzee DNA (see Methods), and are shown in Fig. 4 . Both the yin and yang haplotypes are significantly different from the ancestral haplotype, sharing only 51.4% and 48.6% identity by state, respectively. The macaque, orangutan and chimpanzee haplotypes are also shown in Fig. 4 and are generally similar to the ancestral haplotype. 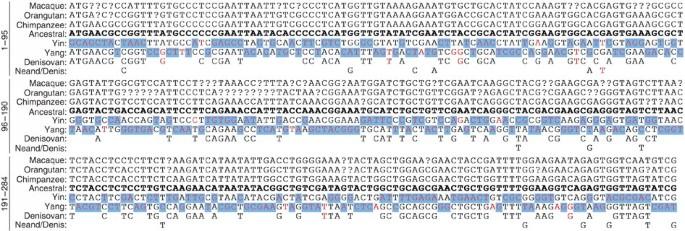Figure 4: Haplotype comparisons. Reference alleles from the UCSC Genome Browser database are shown for macaque, orangutan and chimpanzee. The ancestral alleles are supplied from NCBI’s dbSNP website (see Methods). Red font indicates variation from these ancestral alleles for the yin and yang haplotypes, the haplotype drawn from the individual from the Denisovan fossil site28and the 15 SNP alleles representing several Neandertal and the Denisovan individual (Neand/Denis, see Methods). All 125 identified genotypes for the Denisovan haplotype are homozygous for the allele shown and this haplotype matches the yang haplotype at all 125 sites. However, it is also highly similar to the ancestral haplotype, with 95.2% of the alleles matching. On the other hand, 11 of the 15 Neand/Denis alleles match the yin alleles, while the remaining four match the ancestral, chimpanzee, orangutan and macaque alleles. All but one of the Neand/Denis alleles match the ancestral haplotype and the derived allele matches the yin haplotype. Note that the variation that defines the yin and yang haplotypes (red font) is predominantly unique as 92.6% of the 284 alleles do not match the Neand/Denis, Denisovan, chimpanzee or orangutan alleles (blue shading). Both the yin and yang haplotypes are dissimilar from the ancestral haplotype, having only about half of the SNP alleles in common, yet these two haplotypes are highly conserved across modern human populations. SeeSupplementary Data Set 1for additional information. Figure 4: Haplotype comparisons. Reference alleles from the UCSC Genome Browser database are shown for macaque, orangutan and chimpanzee. The ancestral alleles are supplied from NCBI’s dbSNP website (see Methods). Red font indicates variation from these ancestral alleles for the yin and yang haplotypes, the haplotype drawn from the individual from the Denisovan fossil site [28] and the 15 SNP alleles representing several Neandertal and the Denisovan individual (Neand/Denis, see Methods). All 125 identified genotypes for the Denisovan haplotype are homozygous for the allele shown and this haplotype matches the yang haplotype at all 125 sites. However, it is also highly similar to the ancestral haplotype, with 95.2% of the alleles matching. On the other hand, 11 of the 15 Neand/Denis alleles match the yin alleles, while the remaining four match the ancestral, chimpanzee, orangutan and macaque alleles. All but one of the Neand/Denis alleles match the ancestral haplotype and the derived allele matches the yin haplotype. Note that the variation that defines the yin and yang haplotypes (red font) is predominantly unique as 92.6% of the 284 alleles do not match the Neand/Denis, Denisovan, chimpanzee or orangutan alleles (blue shading). Both the yin and yang haplotypes are dissimilar from the ancestral haplotype, having only about half of the SNP alleles in common, yet these two haplotypes are highly conserved across modern human populations. See Supplementary Data Set 1 for additional information. Full size image The available Neandertal and Denisovan data also predominantly match the ancestral alleles. Figure 4 displays 15 SNP alleles for three Neandertal and the single individual available from the Denisovan fossil site [25] , [26] (Neand/Denis) that have been typed on the Affymetrix HuOrigin array [27] . The SNP ascertainment approach for the HuOrigin array had a bias for SNPs with matching Denisovan and chimpanzee alleles (see Methods). As shown in Fig. 4 , all but 1 of the 15 matches the chimpanzee and ancestral alleles. In all, 11 of the 15 SNP alleles, including the derived allele, match the yin haplotype. Also shown in Fig. 4 are high-coverage genotypes for the Denisovan individual [28] . In contrast to the Neand/Denis data, all 125 SNPs match the yang haplotype. Although there is no apparent reason to expect a bias in these data, 95.2% of the alleles are identical by state (IBS) with both the ancestral and chimpanzee alleles. This is unexpected as less than half of the yang alleles are IBS with the ancestral alleles. Overall, although the yin–yang genotypic patterns are not conserved across species outside the Homo genus, they are highly conserved across the HapMap populations, with combined frequencies ranging from 0.28 to 0.80 for the pair, as detailed in Fig. 1 . Selection for the yin and yang haplotypes Several lines of evidence suggest the yin and yang haplotypes are under strong positive selection and bear functional importance. First, a series of diverse statistical tests for selection indicate positive selection for the region, as shown in Fig. 5 . The left panel of the figure shows the results for four selection tests computed over four HapMap populations. The right panel shows results for selection tests computed over the 1000 Genomes Project data (released April 2012). The topmost plot on the right represents a selective sweep scan on Neandertal versus human polymorphisms, followed by rank scores for 13 tests for selection [29] (see Methods). Both panels include results from Fay and Wu’s [30] H -test. This test was specifically designed to distinguish between positive selection and background selection by using data from outgroup species. As shown in the figure, the yin–yang interval has a statistically significant H -value. Taken together, these results indicate strong positive selection within the yin–yang region. 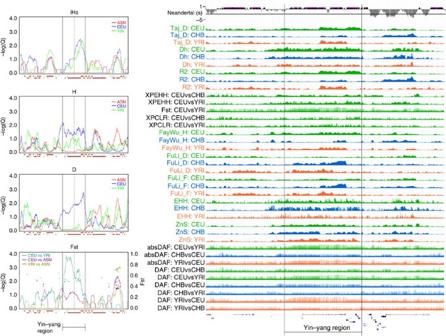Figure 5: Statistical tests for selection. Results from Haplotter22(left) and The 1000 Genomes Selection Browser 1.0 (ref.29) (right). See Methods for descriptions of tests. Left panel displays results for selection tests over a 5-Mb window centred ongephyrinfor four HapMap populations, CEU, YRI, CHB and JPT. The CHB and JPT are combined and labelled as ‘ASN’ in the plots. These plots include Voightet al.’s iHs22, Fay and Wu’sH-test30, Tajima’s D57andFST. Topmost plot on the right side represents a selective sweep scan on Neandertal versus human polymorphisms usingZ-score±variance (Neandertal), followed by rank scores for 13 tests for selection. The rank scores were computed using an outlier approach based on sorted genome-wide scores and peaks represent regions under positive selection29. Included are Tajima’s D (Taj_D)57, Nei’s Dh (Dh)62, Ramos-Onsins and Rozas’R2(R2)59, Sabetiet al.’s XP-EHH* (XPEHH)60, Weir and Cockerham’s pairwiseFST(Fst)64, Chenet al.’s XP-CLR (XPCLR)65, Fay and Wu’sH-test (FayWu_H)30, Fu and Li’s D (FuLi_D)58, Fu and Li’s F (FuLi_F)58, Sabetiet al.’s EHH_average* (EHH)61, Kelly’s ZnS (ZnS)63, Hoferet al.’s absolute ΔDAF (absDAF)66and Hoferet al.’s standard ΔDAF (DAF)66. Asterisk indicates the method was modified by Pybuset al.29Populations are indicated. This image includes modified screen shots fromhttp://hsb.upf.edu/andhttp://haplotter.uchicago.edu/. Figure 5: Statistical tests for selection. Results from Haplotter [22] (left) and The 1000 Genomes Selection Browser 1.0 (ref. 29 ) (right). See Methods for descriptions of tests. Left panel displays results for selection tests over a 5-Mb window centred on gephyrin for four HapMap populations, CEU, YRI, CHB and JPT. The CHB and JPT are combined and labelled as ‘ASN’ in the plots. These plots include Voight et al .’s iHs [22] , Fay and Wu’s H -test [30] , Tajima’s D [57] and F ST . Topmost plot on the right side represents a selective sweep scan on Neandertal versus human polymorphisms using Z -score±variance (Neandertal), followed by rank scores for 13 tests for selection. The rank scores were computed using an outlier approach based on sorted genome-wide scores and peaks represent regions under positive selection [29] . Included are Tajima’s D (Taj_D) [57] , Nei’s Dh (Dh) [62] , Ramos-Onsins and Rozas’ R 2 (R2) [59] , Sabeti et al .’s XP-EHH* (XPEHH) [60] , Weir and Cockerham’s pairwise F ST (Fst) [64] , Chen et al .’s XP-CLR (XPCLR) [65] , Fay and Wu’s H -test (FayWu_H) [30] , Fu and Li’s D (FuLi_D) [58] , Fu and Li’s F (FuLi_F) [58] , Sabeti et al .’s EHH_average* (EHH) [61] , Kelly’s ZnS (ZnS) [63] , Hofer et al .’s absolute ΔDAF (absDAF) [66] and Hofer et al .’s standard ΔDAF (DAF) [66] . Asterisk indicates the method was modified by Pybus et al . [29] Populations are indicated. This image includes modified screen shots from http://hsb.upf.edu/ and http://haplotter.uchicago.edu/ . Full size image It is worth noting that Nielsen et al . [31] found that gephyrin showed no evidence for positive selection ( P -value=1.0) in the coding regions of the gene. Their calculations were specifically based on the ratio of non-synonymous to synonymous mutations within coding regions. In view of the strong selection pressure in the host genomic region, but not on gephyrin exons, it follows that selection pressures may be acting on functional elements within noncoding regions. Second, the size, composition and geographic distribution of yin and yang haplotypes indicate rapid evolution suggestive of strong positive selection. Although the 284 identified SNPs have 0 IBS between the yin and yang pair, the appearance of these haplotypes across 11 diverse populations must be identity by descent for each haplotype, due to the identical states of hundreds of SNP alleles. Recall that the yin haplotype is prominent in European populations, yang is prominent in African populations and Asian populations have nearly equal proportions. This observation, along with the assumption that the haplotypes are identical by descent, suggests that the Asian occurrences arose via gene flow or admixture. It follows that more than 100 nucleotide mutations became fixed for each of the two haplotypes after their split from each other and before their migration to Asia. Such rapid evolution is indicative of strong selection. Surprisingly, these mutations remain generally fixed in these haplotypes in modern populations and all of the intermediate haplotypes that arose between the initial split and fixed states have low frequencies or have disappeared entirely. Third, the unusual recombination patterns in this region support selection favouring the yin and yang haplotypes. A close examination of Figs 1 , 2 , 3 suggests that recombinants comprising both a yin and a yang parental haplotype are generally rare, in particular within gephyrin and upstream from this gene. Such a recombinant would appear as a horizontal bar comprising blocks that are shown as two different colours in Fig. 1 . As shown in Fig. 2 , 9 of the 340 CHB and JPT haplotypes have between 10% and 90% yin/yang compositions; 6 of these represent yin–yang recombinants and 3 represent intermediate yin or yang haplotypes with >10% mutational variations. Indeed, the prevalence of each of the distinct yin and yang haplotypes, despite strong coexistence and recombination opportunities, indicates very low recombination events between yin and yang haplotypes. However, as shown in Fig. 6 , previous analyses of this region provided by the HapMap Consortium ( http://hapmap.ncbi.nlm.nih.gov/downloads/recombination/ ) reported moderate recombination within the region, including an estimated recombination rate of 9.2 cM Mb −1 at rs10133120 in the 5′-end of gephyrin . Taken together, these results strongly suggest that recombinants comprising two yin haplotypes and/or recombinants comprising two yang haplotypes are more prevalent than recombinants merging yin and yang haplotypes together. This observation suggests that yin and yang haplotypes may have been favourably selected over merged yin and yang recombinants. 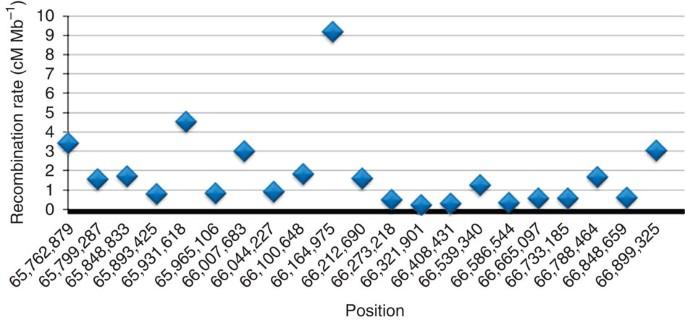Figure 6: Recombination rates. Shown are the recombination rates provided by the HapMap Consortium for the yin–yang region. These rates were computed using the CEU, CHB, JPT and YRI population data. All of these positions are within the yin–yang region and the recombination rate of 9.2 cM Mb−1was estimated at rs10133120 in the 5′-end ofgephyrin. Figure 6: Recombination rates. Shown are the recombination rates provided by the HapMap Consortium for the yin–yang region. These rates were computed using the CEU, CHB, JPT and YRI population data. All of these positions are within the yin–yang region and the recombination rate of 9.2 cM Mb −1 was estimated at rs10133120 in the 5′-end of gephyrin . Full size image It has been estimated that 5% of the human genome is under selection, yet only ~1% of the genome is protein coding [32] , indicating that selection acts on more noncoding than coding regions. Furthermore, transcription is pervasive and ~70%–90% of the human genome is transcribed, producing a vast array of noncoding RNA [33] . Some long noncoding RNA have been documented to play critical regulatory roles. For example, the X-inactivate-specific transcript is vital for inactivating the X chromosome for females by directly binding an epigenetic complex. Closer to protein-coding regions, untranslated regions contain the internal ribosome entry sites and riboswitches that participate in regulation of expression as well as alternative splicing [34] . Furthermore, 3′-untranslated regions host binding sites for microRNAs that inhibit translation [35] . Intronic regions can provide noncoding RNA and are also involved in alternative splicing and transcription regulation [36] . Alternatively, transcription of antisense strands can produce noncoding RNAs involved in a variety of biological roles [37] . The protein-coding regions of gephyrin are highly conserved and its diverse roles are accomplished via regulatory variations. Noncoding elements within its introns and upstream are prime candidates for such regulatory control. Importantly, aberrant regulation of this gene has been associated with a host of complex diseases. Dysfunction in the regulation of gephyrin expression levels and/or isoform production has been implicated for Alzheimer’s disease (AD) [38] , [39] , [40] , epilepsy [9] , [41] , [42] , autism [10] , schizophrenia [10] , [43] , hyperekplexia [13] and chorein deficiency [44] . Gephyrin levels are significantly reduced in AD brains [39] , and the normally strong correlations between gephyrin production and the abundances of the six most common GABA subunits is corrupted in AD brains [38] . It has also been observed that abnormal accumulations of low-molecular-weight gephyrin plaques overlap β-amyloid plaques [40] . Epilepsy is characterized by abnormal excessive excitatory neuronal activities and dysfunction of inhibitory neurons and/or downregulation of inhibitory circuits may be the underlying cause [41] . Gephyrin plays a vital role in inhibitory circuits. Both reduced levels of gephyrin production, as well as the appearance of aberrant gephyrin isoforms, have been observed in epileptogenesis [9] , [41] , [42] . In individuals lacking gephyrin mutations, four aberrant gephyrin isoforms with missing exons have been observed to arise due to cellular stress. These isoforms display dominant negative effects on normal gephyrin in epileptogenesis [9] . Other alternative isoforms have been identified as risk factors for autism and schizophrenia, and may also act as dominant-negative variants [10] . Athanasiu et al . [43] conducted a genome-wide association study of schizophrenia in Norwegian and European samples, and tabulated 32 SNPs in the human genome with the most significant associations. Seven of the 32 are among the yin–yang SNPs, specifically the following: rs1952070, rs6573695, rs17247749, rs17836572, rs1885198, rs6573706 and rs7154017. Overall, the associations of gephyrin regulation with a half-dozen complex diseases strongly motivate the need to understand the genetic machinery driving the diverse manifestations of this highly conserved gene. We present a remarkably long yin–yang haplotype pair spanning the noncoding regions of gephyrin . This genetic phenomenon is more than an order of magnitude larger than any previously reported yin–yang pair and is prevalent across global human populations. Despite the conservation of these haplotypes across human populations, both are highly dissimilar to their common ancestral haplotype, suggesting they are the result of two divergent human-specific evolutionary paths. We advance this hypothesis by reporting several independent lines of evidence supporting selection for the two haplotypes. Taken together, this research lays the groundwork for a deep understanding of the regulatory control of gephyrin . It is not clear how this genetic anomaly arose. Mutation and recombination have created vast amounts of haplotype diversity in many species, including humans. Previous reports have suggested that human-specific traits evolved primarily due to positive selection in noncoding regions involved in the regulation of genes [45] , [46] , [47] . The most eminent of these characteristics is the human brain, with its increased size and enhanced cognition, and it has been demonstrated that selection acting on noncoding regions is predominantly associated with neural development, whereas selection acting on protein-coding regions is associated with immunity, olfaction and male reproduction [47] . In short, it is viable to expect that human-specific adaptations of gephyrin are due to evolution of regulatory mechanisms lying within noncoding regions, in particular those in close proximity. A key question follows: why would two extremely divergent paths arise during such adaptation? One possibility is a chromosomal inversion resulting with a lack of recombination between the original and inverted variant. In such an event, the original and inverted haplotypes would evolve independently. Strong positive selection could drive the evolution of a single high-frequency haplotype for each group. Several systematic searches for inversions have been conducted over the human genome [48] , [49] , [50] . The most recent investigation mapped 6.1 million clones to distinct genomic positions for eight HapMap individuals (four YRI, two CEU, one CHB and one JPT) and identified 224 inversions [50] . One of these is a 31.1-kb inversion in FUT8 , which is 763 kb upstream from gephyrin . However, none of the three studies identified an inversion in the yin–yang region. Another possible impetus for this pattern could be incompatible mutations: that is, two independent mutations each possess a selective advantage individually, but the combination of the two mutations reduces fitness. For example, each of the mutations could increase the expression of a particular gene in a beneficial manner, but together they may produce deleteriously high expression. Selection would favour haplotypes possessing either mutation and recombinants possessing both or neither mutation would become rare. Over time, the two haplotypes bearing each of the original mutations would evolve in distinct manners. At least one other alternate mechanism could have led to the extreme divergence of the yin and yang haplotypes: convergent evolution in isolated ancient populations followed by gene flow [51] . Opportunities for such events have been common throughout human history. For example, recent sequencing of fossil DNA has led to an estimate that modern non-African populations may possess ~1.5%–2.1% Neandertal DNA [52] . DNA related to the single individual found at Denisova is also found in modern island Southeast Asia and Oceania populations, with modern Papuans possessing 6% of their DNA closely related to the Denisovan individual’s DNA [28] . As shown in Fig. 4 , the Neandertal and Denisovan genotypes are highly similar to the ancestral haplotype. However, in addition to the small number of Neandertal genotypes, another weakness of this analysis is that the currently available data are based on few individuals. Increased sample size, increased marker density and further investigations, such as comparisons with nuclear DNA from the 300,000-year-old hominins from Sima de los Huesos [53] when it becomes available, are needed to determine the likelihood that ancient admixture lies at the root of this yin–yang. All of the described hypothetical mechanisms are likely to exhibit differential recombination as is observed for the gephyrin yin–yang pair. The recombination rate among yin haplotypes and the rate among yang haplotypes appear substantially higher than the rate between yin and yang parental haplotypes. Selection is likely to be the strongest for chromosomal inversions, as a recombination event between yin and yang haplotypes results with too few or too many copies of genes upstream and downstream from the cross-over point and general abolition of a gene spanning this point. The existence of recombinants, including those with cross-over points within gephyrin , casts doubt that an inversion underlies this anomaly. On a different note, a test for differential recombination might prove to be a valuable tool for assessing functionality of other yin–yang haplotype pairs previously identified and those to be mapped in the coming years. In general, if the yin and yang haplotypes are not functional, this type of differential recombination across coexisting haplotypes would be improbable. The forces that produced this phenomenon, as well as the biological implications of its presence, invite exploration of an evolutionary ‘road less travelled’ that produced two highly divergent, and uniquely human, genetic patterns intricately interwoven with the conserved protein-coding regions of gephyrin . These results solicit new questions and provide material for hypotheses generation. Several avenues of future research have appealing potential, a couple of which are highlighted below. With regard to gephyrin in particular, deep sequencing of the yin–yang region for ancient and modern populations could be valuable for discerning molecular-level function as well as providing insights into the historical journeys of the haplotypes. In addition, testing for associations between yin–yang status and various phenotypes could provide valuable knowledge. Candidate phenotypes include transcript isoforms, variations of gene expression and susceptibilities to complex diseases such as epilepsy, autism and schizophrenia, which have been previously shown to be associated with distinct isoforms of gephyrin [9] , [10] . It should be noted that the use of animal models in previous studies of gephyrin might have been confounded and misleading, as both the yin and yang haplotypes are uniquely human. More generally, mapping of additional yin–yang haplotypes within the human genome, and other genomes of interest, may pinpoint genetic mechanisms underlying convergent pathways and/or expose regions undergoing rapid evolution. In addition, when combined with geographic distributions, these patterns may provide distinguishable flags for understanding the histories of individuals and populations. Importantly, they may capture valuable features of an individual’s genetic background and their susceptibility to complex traits, perhaps aiding personalized medicine. Looking forward, in addition to increasing our understanding of the human-specific regulation of a vitally important gene, this haplotype pair may serve as a model for studying yin–yang haplotypes and their biological implications for human health and development. HapMap data HapMap bulk data were downloaded from http://hapmap.ncbi.nlm.nih.gov/ . Release HapMap r28, nr.b36 dated 18 Aug 2010 files were downloaded from directory/downloads/genotypes/2010-08_phaseII+III/forward/. Some of the individuals were related, as tabulated here: http://hapmap.ncbi.nlm.nih.gov/downloads/samples_individuals/relationships_w_pops_121708.txt . Data for the children were removed from the data sets, leaving presumably unrelated individuals. For each analysis, the SNPs that were common for all four populations were determined. Next, these data were cleaned to reduce the quantity of missing genotypes as follows. First, the SNPs with at least 50% missing data were removed, then the individuals with at least 50% missing data were removed and finally SNPs with at least 10% missing data were removed. The remaining individuals also had no >10% missing data. In the first analysis, data for four populations were considered: CEU, CHB, JPT and YRI. After removing the children and cleaning, the final data consisted of 1,115,561 autosomal SNPs for 112 CEU, 137 CHB, 113 JPT and 116 YRI, a total of 478 individuals. In the second analysis, data for four different populations were used: GIH with at least three grandparents from Gujarat (the northwest region of the Indian subcontinent), LWK, MKK and TSI. After removing children and cleaning the data, the final data consisted of 1,242,039 autosomal SNPs for 101 GIH, 110 LWK, 143 MKK and 102 TSI, a total of 456 individuals. The three remaining HapMap populations were used to further validate the yin–yang haplotype pair: ASW, CHD and Mexican ancestry in Los Angeles, California. For each population, the genotypes for the 284 SNPs were extracted when available and haplotype frequencies were computed. The genotypes were also plotted for visual inspection ( Fig. 1 ). All of the processed data sets can be obtained by contacting the first author. The 1000 genomes data Chromosome 14 data were downloaded from the 1000 Genomes Project website at ftp://ftp-trace.ncbi.nih.gov/1000genomes/ftp/release/20130502/ on 17 Nov 2014. File ALL.chr14.phase3_shapeit2_mvncall_integrated_v5.20130502.genotypes.vcf.gz, with the last modification noted on 17 Sept 2014, was obtained. A total of 2,504 individuals were genotyped. All markers between 66974125 and 67648525 (GRCh37 coordinates) were extracted, yielding 13,992 markers in the yin–yang region. We extracted the 13,564 biallelic SNPs within this set. Neandertal and Denisova data One Neandertal and two Denisovan data sets were used. The Neand/Denis data for three Vindija Neandertal [25] and one individual from the Denisovan fossil site [26] were downloaded from ftp://ftp.cephb.fr/hgdp_supp10/Harvard_HGDP-CEPH/annotation.txt . The Affymetrix HuOrigin array [27] was used and included 15 SNPs from the yin–yang haplotypes. The data file includes the numbers of high-quality reads for each allele. Only 1 of the 15 SNPs had more than 1 nucleotide state detected for all of the Neandertal and Denisovan reads. SNP rs6573754 (AX-50160621) had one ‘ A ’ and five ‘ G ’s for the Denisovan individual, and three ‘ G ’s for the Neandertal. The ‘ G ’ allele is shown for Neand/Denis in Fig. 4 of the main paper and Supplementary Data Set 1 . Panel 13 of the SNP ascertainment for the HuOrigin array only included SNPs for which the Denisovan allele matched the chimpanzee allele, as this policy facilitated validations [27] . This panel accounted for 20.2% of the original 750,184 SNPs selected, presenting some bias when comparing the 15 Neand/Denis alleles with chimpanzee and ancestral alleles. The second set of Denisovan data was downloaded from UCSC’s Table Browser website ( http://genome.ucsc.edu/cgi-bin/hgTables ) by selecting the ‘Denisova Assembly and Analysis’ group and ‘Denisova Variants’ track from the Human GRCh37/hg19 assembly. The genetic material was drawn from the inner portion of the phalanx of the same individual represented in the Neand/Denis data. A single-stranded library preparation method was used to produce the high-coverage sequence [28] . These data included 125 of the yin–yang haplotype SNPs, three of which were among the 15 SNPs in the Neand/Denis data. BlocBuster BlocBuster is a network approach that uses a multi-faceted, allele-oriented correlation measure [23] , [54] . Briefly, we developed the approach with an aim to identify combinations of correlated alleles that are subjected to genetic heterogeneity. The correlation metric, CCC, is customized for genotype data and appreciates heterogeneity by evaluating four distinct correlations that retain independence between different types of pair-wise correlations. This specification of correlation types is retained in an allele-specific network construction, which increases the network infrastructure yet maintains high efficiency. We determined the CCC threshold using the default method of setting the number of edges in the network equal to the number of SNPs. After preprocessing and cleaning the data, there were 36,542 SNPs in the CEU, CHB, JPT, YRI chromosome 14 data set and 40,820 SNPs in the GIH, LWK, MKK, TSI chromosome 14 data set, and each of the networks contained the corresponding number of edges, representing the most significant CCC correlations for each analysis. Consequently, the average degree of each node in each of the networks was one. The significance of this correlation threshold was tested using permutation trials [23] . After the networks were constructed, groups of nodes that were connected by edges were readily identified, as they were completely isolated from each other. Each of these groups of connected nodes, referred to as blocs, represent a haploid pattern of inter-correlated SNP alleles. The entire pattern of SNP alleles for each of these blocs was tested for possession by each individual. Our open-source code is available at www.blocbuster.org or by contacting the first author. Determination of ancestral allelic similarities Ancestral alleles were compiled from NCBI’s dbSNP webpage ( http://www.ncbi.nlm.nih.gov/projects/SNP/ ). These alleles were supplied by Dr Jim Mullikin of the National Human Genome Research Institute and were determined by comparing human and chimpanzee DNA [55] . A complete list of the alleles for the 284 unique SNPs is supplied in Supplementary Data Set 1 . Haplotype similarities were measured by tallying the numbers of markers that were IBS, a simple yet accurate metric [56] . Selection tests The selection test results were drawn from three sources. First, the Haplotter [22] website ( http://haplotter.uchicago.edu/ ) was used to plot results for four statistics: integrated haplotype score (iHs), H , D and F ST for four HapMap populations (CEU, CHB, JPT and YRI) over a 5-Mb region centred on gephyrin . Voight et al .’s [22] iHs is based on an integration of the extended haplotype homozygosity (EHH) statistic and is designed to capture very recent positive selection. Fay and Wu’s [30] H -statistic detects the effects of hitchhiking on the frequency spectrum as a function of recombination rate. Tajima’s D statistic tests the neutral mutation hypothesis based on the relationship between the average number of nucleotide differences and the number of segregating sites [57] . The fixation index, F ST , is based on Wright’s measure of population differentiation. Second, the 1000 Genomes Selection Browser 1.0 (ref. 29 ) was used to plot the results for a number of statistical tests computed over the 1000 Genomes Project data ( http://www.1000genomes.org/ ) for CEU, CHB and YRI populations. These resequencing data yield higher density information than the original HapMap data and remove most of the SNP ascertainment bias, making them valuable for summary statistics. We included the rank scores, which were computed using an outlier approach based on sorted genome-wide scores [29] . Peaks in the plots represent regions under positive selection. Some of the methods were modified by Pybus et al . [29] and are marked in the following with an asterisk. Three families of statistical tests were included: allele frequency spectrum, LD structure and population differentiation. The allele frequency spectrum family included Tajima’s D (Taj_D) [57] , Fay and Wu’s H (FayWu_H) [30] , Fu and Li’s D (FuLi_D) [58] , Fu and Li’s F (FuLi_F) [58] and Ramos-Onsins and Rozas’ R 2 (R2) [59] . The LD structure family included Sabeti et al .’s XP-EHH* (XPEHH) [60] , Sabeti et al .’s EHH_average* (EHH) [61] , Nei’s Dh (Dh) [62] and Kelly’s ZnS (ZnS) [63] . The population differentiation family included Weir and Cockerham’s pairwise F ST (Fst) [64] , Chen et al .’s XP-CLR (XPCLR) [65] , Hofer et al .’s absolute ΔDAF (absDAF) [66] and Hofer et al .’s standard ΔDAF (DAF) [66] . Third, we used selection statistics generated by Nielsen et al . [31] , which were determined by comparing synonymous and non-synonymous mutations within coding regions. More specifically, the ratio of non-synonymous substitutions per non-synonymous site to synonymous substitutions per synonymous site was tested against the neutral null hypothesis of the ratio being one. Determination of protein conservation The conservation of the gephyrin protein across species was determined using UCSD Signaling Gateway ( http://www.signaling-gateway.org/molecule/ ). Haplotype data The haplotypes for the combined CHB and JPT individuals were identified as follows. First, the SNPs that lie within gephyrin or upstream from gephyrin were extracted from the full HapMap data (positions 65,893,425–66,709,924 from HapMap r28, nr.b36). After removing the five individuals (two CHB and three JPT) with excessive missing data, the SNPs with >5% missing data were discarded, leaving 326 SNPs. Next, the phased haplotypes from the same region for the JPT+CHB individuals were downloaded from the HapMap website ( http://hapmap.ncbi.nlm.nih.gov/downloads/phasing/2009-02_phaseIII/HapMap3_r2/ ). These haplotypes had been inferred using PHASE [67] , [68] and included 170 individuals from the combined CHB and JPT data. We discarded all SNPs that had been identified as having >5% missing values in the original genotype data, leaving a total of 303 phased sites. Haplotype composition plots The haplotype composition plots were constructed using the phased haplotypes for the CHB+JPT populations. These haplotypes were computationally inferred using PHASE [67] . Of the 303 phased sites, 236 represented divergent yin–yang SNPs and the haplotypes comprising these 236 SNP alleles were extracted for the 170 individuals. For each of the 340 phased chromosomes, the percentages of SNP alleles matching the yin and yang haplotypes, respectively, were computed. Genotype heat maps The genotype values for SNPs in the yin–yang region were plotted for visual inspection ( Figs 1 and 3 ). Individuals (rows) were reordered, to place similar individuals near each other. We used our rearrangement clustering method, TSP+ k [69] for this reordering. Briefly, the genotype values for the SNPs for each pattern were extracted from the data and converted to an instance of the Traveling Salesman Problem (TSP) [70] in which each individual was represented as a city. We inserted a dummy city to provide a natural break to the circular TSP tour and determined the ordering of the cities using an iterated Lin–Kernighan local search as implemented by Applegate, Bixby, Chvatal and Cook in the Concorde package ( http://www.math.uwaterloo.ca/tsp/concorde/index.html ). The individuals were reordered using this solution and the genotypes were colour encoded with dark blue, light blue, red and white, representing homozygote for the identified allele, heterozygote, homozygote for the alternate allele and missing data, respectively. How to cite this article: Climer, S. et al . Human gephyrin is encompassed within giant functional noncoding yin–yang sequences. Nat. Commun. 6:6534 doi: 10.1038/ncomms7534 (2015).